A phospholipid uptake system in the model plantArabidopsis thaliana Plants use solar energy to produce lipids directly from inorganic elements and are not thought to require molecular systems for lipid uptake from the environment. Here we show that Arabidopsis thaliana Aminophospholipid ATPase10 (ALA10) is a P4-type ATPase flippase that internalizes exogenous phospholipids across the plasma membrane, after which they are rapidly metabolized. ALA10 expression and phospholipid uptake are high in the epidermal cells of the root tip and in guard cells, the latter of which regulate the size of stomatal apertures to modulate gas exchange. ALA10 -knockout mutants exhibit reduced phospholipid uptake at the root tips and guard cells and are affected in growth and transpiration. The presence of a phospholipid uptake system in plants is surprising. Our results suggest that one possible physiological role of this system is to internalize lysophosphatidylcholine, a signalling lipid involved in root development and stomatal control. P4-ATPases (flippases) are unique to eukaryotes, where they are present in the plasma membrane and membranes of the secretory pathway [1] , [2] , [3] , [4] . At the expense of ATP, these enzymes actively flip phospholipids from one side of the membrane bilayer to the other to create phospholipid asymmetry between the two membrane leaflets. Such local phospholipid imbalances are hypothesized to foster membrane budding, which is the first step in membrane vesicle formation and a hallmark of the secretory and endocytic pathways [1] , [5] . The active unit of flippases is a heterodimeric αβ complex: while the P4-ATPase constitutes the catalytic α-subunit, the β-subunit exhibits chaperone-like features and belongs to the Cdc50 family [1] , [3] . The P4-ATPases present in Saccharomyces cerevisiae are well characterized, and are involved in phospholipid translocation and vesiculation. In total, S. cerevisiae harbours five members of this family [6] , namely Neo1p (Neomycin resistant 1) [7] , Drs2p (Deficient for Ribosomal Subunit 2) [8] , Dnf1p (Drs2p/Neo1p family), Dnf2p and Dnf3p [9] . Neo1p is the only essential member [7] of the family while the four remaining members can be knocked out in all combinations, except for all four at once, without leading to lethality [9] . Whereas Neo1p is located in the early endosome [10] , Drs2p and Dnf3p occur in the trans-Golgi network [9] , and Dnf1p and Dnf2p are both located at the plasma membrane [9] . Likewise, several of the 14 P4-ATPases identified in humans [11] have been linked to phospholipid translocation and have been localized to the plasma membrane, the Golgi, and early endosomes [12] . In Arabidopsis thaliana , P4-ATPases constitute the largest subfamily of P-type ATPase pumps [13] . The catalytic α-subunit family consists of 12 members in A. thaliana , AminophosphoLipid ATPase1-12 (ALA1-12) [13] , [14] . A smaller family of β-subunits, ALA Interacting Subunits1-5 (ALIS1-5) [15] , assists in the maturation of α-subunits and their exit from the ER [16] . Some of these plant ALA proteins have been characterized. ALA1, the first member of this family to be identified [14] , localizes to the plasma membrane; however, its biological function and the identity of its transported substrate remain unknown [17] . ALA2 flips phosphatidylserine (PS) across the lipid bilayer in the endosomal system [16] and ALA3 is a broad-specificity phospholipid flippase expressed in the Golgi apparatus, where it contributes to the formation of secretory vesicles [15] . ALA6 and ALA7 have a high degree of functional redundancy and are important for pollen fitness [18] . Nine of the 12 P4-ATPases present in A. thaliana , ALA4-12, show high sequence similarity to each other (>75% identity) and form an apparent monophyletic cluster [13] . The existence of multiple closely related isoforms suggests that these isoforms have important redundant functions and/or are differentially controlled in different cells under different conditions. Indeed, ALA6 and ALA7 have been reported to have a high degree of functional redundancy [18] . Such redundancy complicates genetic analyses and might explain why genes encoding these isoforms have not hitherto appeared in mutant screens. The P4-ATPases from A. thaliana , S. cerevisiae , Homo sapiens and Caenorhabditis elegans have been phylogenetically divided into six classes, with Class 1a including yeast Drs2p and all A. thaliana P4-ATPases except ALA1 and ALA2 (ref. 19 ). In an extensive re-examination of phylogenetic relationships amongst P4-ATPases, we find that ALA3–10 group within a distinct monophyletic class, which consists exclusively of plant proteins. In an attempt to uncover the functions of genes within this class, we selected ALA10 as a representative protein. Large-scale proteomic studies suggest that ALA10 exists as a phosphoprotein at the plasma membrane [20] , [21] . In animal cells, P4-ATPases at this location constantly remove PS from the outer plasma membrane leaflet, which protects cells, as macrophages engulf cells with this phospholipid exposed at their surface [22] . Such a function is unlikely to be required in plants and it is unclear what role a plasma membrane P4-ATPase would fulfil in plants, although PS may also be exposed at the surface of apoptotic plant cells [23] . Here we confirm the localization of ALA10 to the plasma membrane and show that it facilitates internalization of externally applied phospholipids. Although the lipid specificity of ALA10 is broad, our results suggest that ALA10 plays a specific role in the uptake of lysophosphatidylcholine (lysoPC), a signalling lipid involved in plant development. ALA10 belongs to a plant-specific class of P4-ATPases To obtain a first clue as to the function of ALA10, we investigated its relationship to P4-ATPases present in organisms other than A. thaliana . We generated phylogenetic trees harbouring 162 sequences from a total of 27 genomes representing different stages in the evolution of plants, fungi and animals. The tree with the highest likelihood is shown in Fig. 1 . The phylogenetic tree identified seven monophyletic clusters including 12 kingdom-specific clades with three clades being specific to plants, four to fungi and five to animals. Among the monophyletic clusters, six roughly corresponded to Classes 1–6 in the previous classification [19] , even though in our analysis Class 3 (including S. cerevisiae Dnf1p and Dnf2p) and Class 5 grouped together in a monophyletic cluster. A major cluster representing plant sequences only (here named Class 7) was novel and comprised sequences from green algae (a single gene only in picoplankton species), mosses, clubmosses and flowering plants (including A. thaliana ALA3-10). We conclude that Class 7 P4-ATPases are a hallmark of plants and that the ancestor of ALA10 was present in the first green alga but underwent extensive gene duplication in land plants. The phylogenetic relationship between clusters was less clear. Only Class 2 (including S. cerevisiae Neo1p) appeared as a clear monophyletic group distinct from all other P4-ATPases, whereas the evolutionary connection between other classes could not be identified with statistical certainty as evidenced in a bootstrap consensus tree inferred from 500 replicates, in which branches reproduced in <50% of bootstrap replicates were collapsed ( Supplementary Fig. 1 ). Thus, we were unable to confirm the previous suggestion that ALA10 (Class 7) shares a common origin with S. cerevisiae Drs2p (Subclass 1a) [19] , the founding member of the P4-ATPase family. 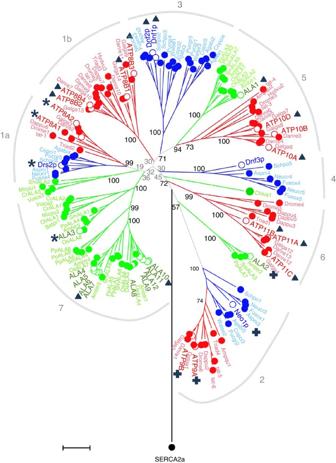Figure 1: Phylogenetic analysis of the P4-ATPase protein family of plant, fungal and animal sequences demonstrates the presence of classes, several of which are kingdom specific. The tree with the highest log likelihood (−92499.4933) inferred from a maximum likelihood analysis as described in the Methods section is shown. The tree is drawn to scale, with branch lengths measured in the number of substitutions per site. Numbers at the nodes reflect the percentage of 500 replicate bootstrap trees, which resolve the clade at the endpoints of that branch. P4-ATPases are phylogenetically split into seven Classes (numbered 1–7) among which Class 1 is further divided into two subclasses, a and b. ALA10 belongs to Class 7, which is specific to plants. Database accession numbers are given in the Methods section. Plantae: ALA, P4-ATPases fromArabidopsis thaliana; Ambtr,Amborella trichopoda; Batpr,Bathycoccus prasinos; Chlva,Chlorella variabili;Cr,Chlamydomonas reinhardtii; Micpu,Micromonas pusilla; Pp,Physcomitrella patens; Os,Oryza sativa; Ot,Ostreococcus tauri; Sm,Selaginella moellendorffii; and Volca,Volvox carteri; Fungi: Drs2p, Dnf1p, Dnf2p, Dnf3p, and Neo1p, P4-ATPases fromSaccharomyces cerevisiae; Agabi,Agaricus bisporus; Aspi,Aspergillus nidulans; Copci,Coprinopsis cinerea; Fo,Fusarium oxysporum; Neucr,Neurospora crassa; Pucgr,Puccinia graminis; Schpo,Schizosaccharomyces pombe; and Walse,Wallemia sebi; Animalia: ATP8-11, P4-ATPases fromHomo sapiens;Galga,Gallus gallus;Danre,Danio rerio;Dappu,Daphnia pulex; Drome,Drosophila melanogaster;tat1-5, P4-ATPases fromCaenorhabditis elegans;Hydvu,Hydra vulgaris;Ampqu,Amphimedon queenslandica; Triad,Trichoplax adhaerens; and SERCA2a, P2-type (non-P4) ATPase fromOryctolagus cuniculus(P05023). Intracellular localization of P4-ATPases fromA. thaliana,S. cerevisiaeandH. sapiens12is indicated as follows: triangles, plasma membrane; asterisks,trans-Golgi apparatus; crosses, endomembranes (endosomes, early endosomes,trans-Golgi apparatus). Blue, fungi isoforms; green, plantae isoforms; and red, animalia isoforms. Scale bar, 0.2 amino-acid substitution per site. Figure 1: Phylogenetic analysis of the P4-ATPase protein family of plant, fungal and animal sequences demonstrates the presence of classes, several of which are kingdom specific. The tree with the highest log likelihood (−92499.4933) inferred from a maximum likelihood analysis as described in the Methods section is shown. The tree is drawn to scale, with branch lengths measured in the number of substitutions per site. Numbers at the nodes reflect the percentage of 500 replicate bootstrap trees, which resolve the clade at the endpoints of that branch. P4-ATPases are phylogenetically split into seven Classes (numbered 1–7) among which Class 1 is further divided into two subclasses, a and b. ALA10 belongs to Class 7, which is specific to plants. Database accession numbers are given in the Methods section. Plantae: ALA, P4-ATPases from Arabidopsis thaliana ; Ambtr, Amborella trichopoda ; Batpr, Bathycoccus prasinos ; Chlva, Chlorella variabili ; Cr , Chlamydomonas reinhardtii ; Micpu, Micromonas pusilla ; Pp, Physcomitrella patens ; Os, Oryza sativa ; Ot, Ostreococcus tauri ; Sm, Selaginella moellendorffii ; and Volca, Volvox carteri ; Fungi: Drs2p, Dnf1p, Dnf2p, Dnf3p, and Neo1p, P4-ATPases from Saccharomyces cerevisiae ; Agabi, Agaricus bisporus ; Aspi, Aspergillus nidulans ; Copci, Coprinopsis cinerea ; Fo, Fusarium oxysporum ; Neucr, Neurospora crassa ; Pucgr, Puccinia graminis ; Schpo, Schizosaccharomyces pombe ; and Walse, Wallemia sebi ; Animalia: ATP8-11, P4-ATPases from Homo sapiens; Galga, Gallus gallus; Danre, Danio rerio; Dappu, Daphnia pulex ; Drome, Drosophila melanogaster; tat1-5, P4-ATPases from Caenorhabditis elegans; Hydvu, Hydra vulgaris; Ampqu, Amphimedon queenslandica ; Triad, Trichoplax adhaerens ; and SERCA2a, P2-type (non-P4) ATPase from Oryctolagus cuniculus (P05023). Intracellular localization of P4-ATPases from A. thaliana , S. cerevisiae and H. sapiens [12] is indicated as follows: triangles, plasma membrane; asterisks, trans -Golgi apparatus; crosses, endomembranes (endosomes, early endosomes, trans -Golgi apparatus). Blue, fungi isoforms; green, plantae isoforms; and red, animalia isoforms. Scale bar, 0.2 amino-acid substitution per site. Full size image When the known subcellular localizations of characterized P4-ATPase members from the model organisms A. thaliana , S. cerevisiae and H. sapiens were plotted in the phylogenetic tree, members of Subclass 1b and Classes 3, 5 and 6 were found to localize to the plasma membrane, whereas those of Subclass 1a and Class 2 appeared specific to the Golgi apparatus and endomembranes ( trans -Golgi network, early endosomes and endosomes), respectively ( Fig. 1 and Supplementary Fig. 1 ). This suggests that membrane localization is class specific. However, the localization pattern of the newly identified Class 7 P4-ATPases was less clear. ALA10 has been identified in large-scale phosphoproteomics studies of the plasma membrane [20] , [21] , ALA6 has been localized to the plasma membrane but also to highly mobile endomembrane structures [18] , whereas ALA3, in an outgroup of its own, has been localized to the Golgi apparatus [15] . This prompted us to investigate the localization of ALA10 in more detail. ALA10 is a plasma membrane protein To investigate the membrane localization of ALA10, we cloned ALA10 and generated an amino-terminal (N-terminal) fusion of green fluorescent protein (GFP) to ALA10 ( GFP-ALA10 ) for transient expression in tobacco epidermal cells. When this construct was co-expressed with the ER retention signal HDEL fused to yellow fluorescent protein (YFP), a clear ER overlay of the two signals was observed ( Fig. 2a ). By contrast, when co-expressing GFP-ALA10 with ALIS1 (as well as ALIS3 and ALIS5) fused to YFP, the fluorescence of both proteins was observed in the periphery of cells ( Fig. 2b , top panel; Supplementary Fig. 2a ). When cells co-expressing GFP-ALA10 and an ALIS-YFP were plasmolysed by osmotic shock, the fluorescent signal retracted from the cell wall, indicating that ALA10 is indeed localized to the plasma membrane ( Fig. 2b , Supplementary Fig. 2a ). As expected, this retraction was not complete, as the plasma membrane still remained attached at some points to the cell wall, through membrane structures known as Hechtian strands. The plasma membrane localization appeared not to be an artefact of overexpression, as the only fluorescent signal present in selected cells expressing GFP-ALA10 with an untagged ALIS (chosen for being at the lower limit of detection for the GFP signal) was in the contour of the cell and surrounding the nucleus ( Fig. 2c , Supplementary Fig. 2b ). Furthermore, no fluorescence was found to wrap around the nucleus, as would be expected if overexpressed membrane protein accumulated in the ER. 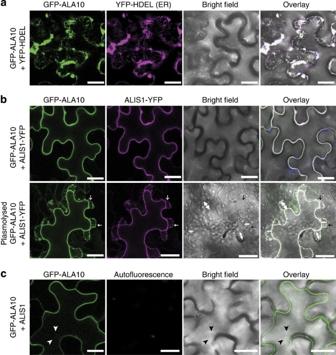Figure 2: ALA10 localizes to the plasma membrane when expressed in tobacco. (a) GFP-ALA10 was transiently expressed in tobacco epidermal cells, in concert with a YFP fusion of the HDEL ER retention signal. The GFP and YFP signals overlapped. (b) GFP-ALA10 was transiently expressed in tobacco epidermal cells, in the presence of ALIS1-YFP. The proteins co-localized at a membrane structure that follows the contour of the cell. In plasmolysed cells, bidirectional arrows mark the position of the plasma membrane with respect to the cell wall at places where the membrane has contracted due to cell shrinkage. Connections between the plasma membrane and the cell wall (Hechtian strands) are marked by directional arrows. (c) GFP-ALA10 was transiently expressed in tobacco epidermal cells, in the presence of untagged ALIS1. To avoid artefacts due to overexpression, only cells with low GFP signal were visualized. Indicative of plasma membrane localization, GFP-ALA10 localizes to a membrane structure that follows the contour of the cell but not the nucleus (arrowhead). Scale bar, 25 μm. Figure 2: ALA10 localizes to the plasma membrane when expressed in tobacco. ( a ) GFP-ALA10 was transiently expressed in tobacco epidermal cells, in concert with a YFP fusion of the HDEL ER retention signal. The GFP and YFP signals overlapped. ( b ) GFP-ALA10 was transiently expressed in tobacco epidermal cells, in the presence of ALIS1-YFP. The proteins co-localized at a membrane structure that follows the contour of the cell. In plasmolysed cells, bidirectional arrows mark the position of the plasma membrane with respect to the cell wall at places where the membrane has contracted due to cell shrinkage. Connections between the plasma membrane and the cell wall (Hechtian strands) are marked by directional arrows. ( c ) GFP-ALA10 was transiently expressed in tobacco epidermal cells, in the presence of untagged ALIS1. To avoid artefacts due to overexpression, only cells with low GFP signal were visualized. Indicative of plasma membrane localization, GFP-ALA10 localizes to a membrane structure that follows the contour of the cell but not the nucleus (arrowhead). Scale bar, 25 μm. Full size image ALA10 is expressed in roots and stomatal guard cells To analyse the tissue-specific expression of ALA10 , we cloned the promoter region of the gene, fused it with the coding region of the reporter gene β-glucuronidase ( GUS ), and stably introduced the construct into A. thaliana . Reporter gene staining was strong in the roots of transgenic seedlings expressing GUS under the control of the ALA10 promoter, and ended abruptly at the junction with the hypocotyl ( Fig. 3a ). In cotyledons, staining was confined to stomatal guard cells and displayed considerable variability in intensity ( Fig. 3b ). At the root tip, staining was strong ( Fig. 3c–e ). The reporter gene was expressed in the epidermal cell layer exposed to the growth medium ( Fig. 3e ). 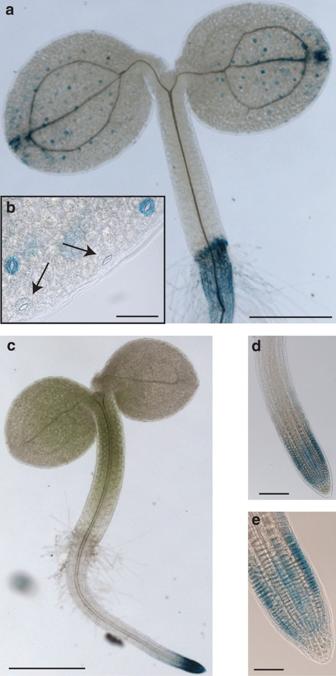Figure 3:ALA10is expressed in guard cells and root epidermal cells. Visualization ofALA10promoter-GUS expression in 5-day-oldA. thalianaseedlings after 12 h (a,b) or 40 min (c–e) of tissue staining. (a) Aerial tissues. (b) Guard cells of the cotyledons. (c) Full view of seedling. (d) Root tip. (e) Magnification of root tip in (d). Arrows indicate the position of unstained guard cells. Scale bars, (a,c) 0.5 mm; (b,e), 0.05 mm; (d), 0.1 mm. Figure 3: ALA10 is expressed in guard cells and root epidermal cells. Visualization of ALA10 promoter-GUS expression in 5-day-old A. thaliana seedlings after 12 h ( a , b ) or 40 min ( c – e ) of tissue staining. ( a ) Aerial tissues. ( b ) Guard cells of the cotyledons. ( c ) Full view of seedling. ( d ) Root tip. ( e ) Magnification of root tip in ( d ). Arrows indicate the position of unstained guard cells. Scale bars, ( a , c ) 0.5 mm; ( b , e ), 0.05 mm; ( d ), 0.1 mm. Full size image ALA10 internalizes lysoPC and glycerophospholipids in yeast To study the biochemical function of ALA10, we co-expressed ALA10 with ALIS1 , ALIS3 or ALIS5 under the control of a galactose-inducible promoter and with an N-terminally located RGSH 10 or RGSH 6 tag for detection, in a S. cerevisiae mutant (ZHY709) that lacks the endogenous plasma membrane P4-ATPases Dnf1p and Dnf2p, as well as the Golgi-localized P4-ATPase Drs2p [9] ( Fig. 4a , Supplementary Fig. 3a ). As controls, we co-expressed ALA2 with ALIS5 and ALA3 with ALIS1, which are known to form complexes with each other [15] , [16] . All ALA and ALIS proteins were detectable in yeast microsomal membranes ( Fig. 4b , Supplementary Fig. 3b ) and, as exemplified by the GFP-ALA10 protein, all ALA+ALIS complexes reached the plasma membrane ( Fig. 4c , Supplementary Fig. 3c ). Papuamide B is a depsipeptide that binds to PS exposed at the cell surface and causes cell death [16] . When papuamide B was present in the growth medium, ZHY709 cells failed to grow; however, growth was recovered in the presence of ALA10+ALIS , demonstrating that an active ALA10 complex is able to remove PS from the outer leaflet of the plasma membrane ( Fig. 4a , Supplementary Fig. 3a ). A catalytically inactive mutant of ALA10, in which the conserved P-type phosphorylation residue (Asp430) is mutagenised to Asn ( ala10 ), could not complement the mutant yeast strain in the presence of papuamide B ( Fig. 4a ), whereas, like ALA10+ALIS1 , both the ALA2+ALIS5 and ALA3+ALIS1 combinations could ( Fig. 4a ). Duramycin binds exclusively to surface-exposed phosphatidylethanolamine (PE) and thus causes cell death of ZHY709 cells ( Fig. 4a ) [16] . In the presence of this compound, ALA10+ALIS and ALA3+ALIS1 complemented the ZHY709 mutant, whereas cells expressing ALA2+ALIS5 were not viable ( Fig. 4a , Supplementary Fig. 3a ), indicating that ALA10 and ALA3 transport PE, whereas ALA2 does not. Miltefosine (hexadecylphosphocholine) is a choline-containing lysoPC analogue that is toxic only after uptake across the plasma membrane [24] . Wild-type yeast is sensitive to miltefosine, whereas ZHY709 is not ( Fig. 4a ). In the presence of the ALA10+ALIS complexes, mutant cells became sensitized to miltefosine, whereas cells expressing ALA2+ALIS5 or ALA3+ALIS1 remained tolerant ( Fig. 4a , Supplementary Fig. 3a ). Thus, ALA10 internalizes miltefosine, whereas ALA2 and ALA3 do not. This activity was also apparent when ALA10 was co-expressed with ALIS3 or ALIS5, and when ALA10 was replaced with GFP-ALA10, indicating that the GFP fusion used previously for localization in plant cells is also functional in yeast ( Fig. 4a , Supplementary Fig. 3a ). Notably, the cold-sensitive phenotype of the drs2 ZHY709 mutant could not be complemented by the ALA10+ALIS combinations, indicating that ALA10 does not have similar functions to the Golgi-localized Drs2p ( Fig. 4a , Supplementary Fig. 3a ). 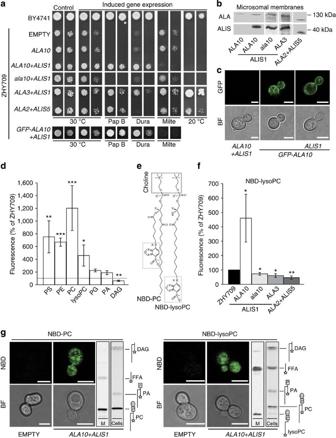Figure 4:ALA10complements the phenotypes of the P4-ATPase-deficient yeast strain ZHY709 and translocates NBD-PS, -PE, -PC and lysoPC. (a) Functional complementation of a P4-ATPase-deficient yeast strain (ZHY709) expressing wild-typeALA10(RGSH10-ALA10) and mutantala10(ala10D430N) in combination with the β-subunitALIS1(RGSH6-ALIS1). Yeast strain BY4741 (wild type) and ZHY709 transformed with empty plasmids were used as a positive and negative control, respectively. Yeast strains were grown at 30 °C on glucose- (control) or galactose-containing (induced gene expression) plates supplemented with papuamide B (Pap B), duramycin (Dura), and miltefosine (Milte) or on plates incubated at 20 °C, as indicated. The experiment was repeated at least three times with identical results. (b) Immunoblot illustrating the expression of P4-ATPases and co-expressed β-subunits in yeast microsomal membranes (Anti-RGSHis). (c) Subcellular localization of GFP-ALA10 in the presence and absence of RGSH6-ALIS1. BF, bright field. Scale bar, 5 μm. (d) ZHY709 yeast cells expressingALA10+ALIS1were labelled with the indicated NBD-lipids and analysed by flow cytometry. Accumulation of NBD-lipids is shown as a percentage of fluorescence intensity relative to ZHY709 (dotted line), arbitrary values corresponding to 100% are given for all lipids in the Methods section. Data represent means±s.d. (n=3-17). ***P≤0.001, **P≤0.01 and *P≤0.05, significantly different with respect to ZHY709 according to Student’st-test. (e) Chemical structure of NBD-PC and -lysoPC; black box, choline head group; grey box, NBD. (f) NBD-lysoPC accumulation in ZHY709 cells transformed with different plant P4-ATPases and their respective β-subunits. Data represent means±s.d. (n=3–4). **P≤0.01 and *P≤0.05, significantly different with respect to ZHY709 according to Student’st-test. (g) ALA10+ALIS1-dependent NBD-PC and -lysoPC uptake and analysis of metabolized lipids. Cells expressing ALA10+ALIS1 or containing empty vector (EMPTY) were incubated with NBD-lipids for 30 min before imaging by fluorescence (NBD) or bright field (BF) microscopy (left). Scale bar, 5 μm. For analysis by thin-layer chromatography (right), lipids were extracted from labelled cells (Cells) and their medium (M). Lipid structures are given to the right in each figure (circle, choline; square, phosphate group; star, NBD group). Figure 4: ALA10 complements the phenotypes of the P4-ATPase-deficient yeast strain ZHY709 and translocates NBD-PS, -PE, -PC and lysoPC. ( a ) Functional complementation of a P4-ATPase-deficient yeast strain (ZHY709) expressing wild-type ALA10 (RGSH 10 -ALA10) and mutant ala10 ( ala10D430N ) in combination with the β-subunit ALIS1 (RGSH 6 -ALIS1). Yeast strain BY4741 (wild type) and ZHY709 transformed with empty plasmids were used as a positive and negative control, respectively. Yeast strains were grown at 30 °C on glucose- (control) or galactose-containing (induced gene expression) plates supplemented with papuamide B (Pap B), duramycin (Dura), and miltefosine (Milte) or on plates incubated at 20 °C, as indicated. The experiment was repeated at least three times with identical results. ( b ) Immunoblot illustrating the expression of P4-ATPases and co-expressed β-subunits in yeast microsomal membranes (Anti-RGSHis). ( c ) Subcellular localization of GFP-ALA10 in the presence and absence of RGSH 6 -ALIS1. BF, bright field. Scale bar, 5 μm. ( d ) ZHY709 yeast cells expressing ALA10+ALIS1 were labelled with the indicated NBD-lipids and analysed by flow cytometry. Accumulation of NBD-lipids is shown as a percentage of fluorescence intensity relative to ZHY709 (dotted line), arbitrary values corresponding to 100% are given for all lipids in the Methods section. Data represent means±s.d. ( n =3-17). *** P ≤0.001, ** P ≤0.01 and * P ≤0.05, significantly different with respect to ZHY709 according to Student’s t -test. ( e ) Chemical structure of NBD-PC and -lysoPC; black box, choline head group; grey box, NBD. ( f ) NBD-lysoPC accumulation in ZHY709 cells transformed with different plant P4-ATPases and their respective β-subunits. Data represent means±s.d. ( n =3–4). ** P ≤0.01 and * P ≤0.05, significantly different with respect to ZHY709 according to Student’s t -test. ( g ) ALA10+ALIS1-dependent NBD-PC and -lysoPC uptake and analysis of metabolized lipids. Cells expressing ALA10+ALIS1 or containing empty vector (EMPTY) were incubated with NBD-lipids for 30 min before imaging by fluorescence (NBD) or bright field (BF) microscopy (left). Scale bar, 5 μm. For analysis by thin-layer chromatography (right), lipids were extracted from labelled cells (Cells) and their medium (M). Lipid structures are given to the right in each figure (circle, choline; square, phosphate group; star, NBD group). Full size image To obtain a more direct measure of phospholipid transport, we used the same yeast system to measure the uptake of fluorescent 7-nitrobenz-2-oxa-1,3-diazole (NBD) acyl-labelled lipid reporters ( Fig. 4d ). In this assay, yeast cells are incubated with NBD-labelled lipids and, following the removal of surface-exposed probe, the remaining fluorescence is assayed [25] . This assay confirmed that the ALA10+ALIS complex internalizes labelled PS, PE and phosphatidylcholine (PC; Fig. 4d , Supplementary Fig. 3d ). In addition, lysoPC, which lacks the acyl chain present at the sn-2 position in PC ( Fig. 4e ), was readily internalized ( Fig. 4d ). To investigate whether ALA10 translocates all types of glycerophospholipids, we analysed the uptake of labelled phosphatidylglycerol (PG) and phosphatidic acid (PA) and found the NBD signal not to be significantly different from background levels ( Fig. 4d , Supplementary Fig. 4a ). Similarly, diacylglycerol (DAG), which lacks a phosphate group present in the other lipids, was not transported into the yeast cells ( Fig. 4d ). There was a marked qualitative difference between ALA10 and the other P4-ATPases examined: neither ALA2 nor ALA3 in complex with an ALIS subunit transported detectable levels of lysoPC, whereas the ALA10+ALIS1 complex did ( Fig. 4f ). Because the size and position of the bulky NBD group might interfere with the integration of the lipid in the membrane ( Fig. 4e ), especially in the case of lysoPC, which has only one acyl chain, the transport rates of natural phospholipids might be different from those labelled with NBD, making it difficult to compare the data quantitatively. However, the results suggest that the ALA10+ALIS complex preferentially transports phospholipids with a choline head group. In ALA10-expressing yeast cells, NBD-labelled PC, PE and PS were detected inside cells, with at least NBD-PC and -PS being metabolized ( Fig. 4g , Supplementary Fig. 4b ). Very low levels of NBD-lysoPC were detected inside the yeast cells ( Fig. 4g ), as it was intracellularly metabolized to NBD-PC, -PA, -DAG and -free fatty acid (FFA) derivatives ( Fig. 4g ). ALA10 internalizes lysoPC and glycerophospholipids in planta The identification of a plant lysoPC transporter was unexpected, and we therefore aimed to investigate whether the lysoPC transport specificity of ALA10 was also evident in its natural environment. To confirm the transport capabilities of ALA10 in planta , we identified three independent T-DNA knockout mutants of ALA10 in A. thaliana and produced homozygous mutant lines, which we named ala10-1 , ala10-5 and ala10-7 , respectively ( Fig. 5a ). When seedlings of wild-type A. thaliana were incubated in a defined medium and NBD-PS, -PE, -PC or -lysoPC was added, the labelled phospholipids were observed inside the epidermal cells of the root tip after ∼ 1 h of incubation and fluorescence continued to increase in the subsequent hours ( Fig. 5b,c , left panel, Supplementary Fig. 5 ). Remarkably, following uptake into the root, labelled PC was rapidly metabolized to PA, DAG and FFA. By contrast, labelled lysoPC was converted into PC, PA, DAG, FFA and other products ( Fig. 5b , right panel). Ground-root controls incubated with the same NBD-lipids demonstrated that formation of some of the lipid species observed inside the plants requires the presence of intact plant tissues. In all three ala10 -knockout lines, the uptake rates of labelled glycerophospholipids were markedly diminished ( Fig. 5c , Supplementary Fig. 5 ). No differences in staining were observed when wild-type and ala10 plants were incubated with the endocytic tracer dye, FM4-64 ( Fig. 5d ), thus ruling out a block in endocytosis as the reason for the reduced lipid uptake in the mutants. We conclude that ALA10 contributes to the root cellular uptake of external PC and lysoPC and also to the uptake of PS and PE, which generally occurs at a slower rate compared to PC and lysoPC. 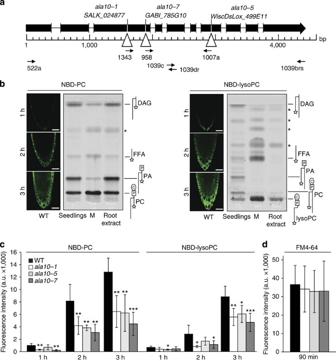Figure 5: NBD-PC and -lysoPC are taken up intoA. thalianaroots in anALA10-dependent manner. (a) Three independentala10-knockout lines (ala10-1,ala10-5andala10-7) were isolated and tested for homozygosity. Numbers under the DNA fragment denote primers used for homozygosity testing. Black boxes, exons; lines, introns; triangles, T-DNA insertion sites. Size onxaxis is given in base pairs (bp). (b) Five-day-old wild-type seedlings were incubated in the presence of NBD-PC or -lysoPC, as indicated. Left, confocal microscopy visualization of NBD fluorescence. Scale bar, 25 μm. Right, after 3 h of NBD-lipid incubation, lipids were extracted from root tissues (Seedlings) and from media (M) and subjected to thin-layer chromatography. Root extract, ground roots incubated with NBD-lipid for 30 min and treated in a similar manner. Asterisks (*), unidentified contaminants already present in the original NBD-lipid stock. Lipid structures are given to the right in each figure (circle, choline; square, phosphate group; star, NBD group). (c) Five-day-oldA. thalianawild-type and mutant seedlings were incubated in the presence of NBD-PC or -lysoPC for 1–3 h before visualization by confocal microscopy and quantification. Data represent means±s.d. (n=5–7 from three biological replicates). (d) Five-day-old seedlings corresponding to the wild-type orala10-knockout lines were incubated in the presence of the endocytic tracker FM4-64 for 90 min before visualization by confocal microscopy and quantification. FM4-64 fluorescence intensity was measured. Data represent means±s.d. (n=22–25 from three biological replicates). ***P≤0.001, **P≤0.01 and *P≤0.05, significantly different with respect to wild type based on Student’st-test. Figure 5: NBD-PC and -lysoPC are taken up into A. thaliana roots in an ALA10 -dependent manner. ( a ) Three independent ala10 -knockout lines ( ala10-1 , ala10-5 and ala10-7 ) were isolated and tested for homozygosity. Numbers under the DNA fragment denote primers used for homozygosity testing. Black boxes, exons; lines, introns; triangles, T-DNA insertion sites. Size on x axis is given in base pairs (bp). ( b ) Five-day-old wild-type seedlings were incubated in the presence of NBD-PC or -lysoPC, as indicated. Left, confocal microscopy visualization of NBD fluorescence. Scale bar, 25 μm. Right, after 3 h of NBD-lipid incubation, lipids were extracted from root tissues (Seedlings) and from media (M) and subjected to thin-layer chromatography. Root extract, ground roots incubated with NBD-lipid for 30 min and treated in a similar manner. Asterisks (*), unidentified contaminants already present in the original NBD-lipid stock. Lipid structures are given to the right in each figure (circle, choline; square, phosphate group; star, NBD group). ( c ) Five-day-old A. thaliana wild-type and mutant seedlings were incubated in the presence of NBD-PC or -lysoPC for 1–3 h before visualization by confocal microscopy and quantification. Data represent means±s.d. ( n =5–7 from three biological replicates). ( d ) Five-day-old seedlings corresponding to the wild-type or ala10 -knockout lines were incubated in the presence of the endocytic tracker FM4-64 for 90 min before visualization by confocal microscopy and quantification. FM4-64 fluorescence intensity was measured. Data represent means±s.d. ( n =22–25 from three biological replicates). *** P ≤0.001, ** P ≤0.01 and * P ≤0.05, significantly different with respect to wild type based on Student’s t -test. Full size image ALA10 affects root growth response to phosphate and lysoPC Genome-wide transcriptional analyses showed that ALA10 transcription is upregulated under phosphate starvation [26] . We confirmed these data by quantitative real-time PCR, which demonstrated a highly reproducible 20% increase of ALA10 transcript levels under these conditions ( Fig. 6a ). To analyse how plant growth is affected by loss of ALA10 , the wild-type and three ala10 mutant lines were grown on phosphate-depleted media for four days. After marking their root tips (day 0), we allowed the plants to grow for another 3 days (day 3). During these days, the primary roots of ala10 plants grew significantly longer than did those of the wild type ( Fig. 6b ). To correlate lysoPC transport by ALA10 with the root growth phenotype, we analysed the effect of lysoPC spotted directly onto the root tip of mutant and wild-type plants on days 0, 1, and 2. In this experiment, only the roots of wild-type plants grew significantly longer in response to treatment with lysoPC, whereas those of the mutant lines did not respond to the lysoPC treatment ( Fig. 6c ). 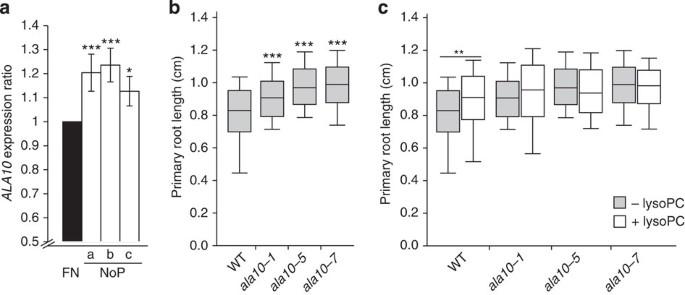Figure 6: Root growth is affected by phosphate starvation and lysoPC application in anALA10-dependent manner. (a)ALA10expression in 7-day-old wild-type seedlings grown on full nutrition (FN) and phosphate depleted (NoP) media was determined by qRT-PCR.a, b and c represent independent biological replicates. Data represent means of technical replicates±s.e.m. (n=6); ***P≤0.001 and *P≤0.05, significantly different from FN grown plants according to REST©70. (b) Primary root length of 7-day-old wild-type andala10seedlings grown on phosphate-depleted media. Data represented as box plot with marked median±s.d. (n=115–165 from three biological replicates); ***P≤0.001, significantly different with respect to wild type (WT) according to Mann–WhitneyU-test. (c) Primary root length of 7- day-old wild-type andala10seedlings grown on phosphate-depleted media with the addition of liquid medium±lysoPC. Data represented as box plot with marked median±s.d. (n=115–165 from three biological replicates); **P≤0.01, significantly different with respect to treatment without lysoPC according to Mann–WhitneyU-test. Figure 6: Root growth is affected by phosphate starvation and lysoPC application in an ALA10 -dependent manner. ( a ) ALA10 expression in 7-day-old wild-type seedlings grown on full nutrition (FN) and phosphate depleted (NoP) media was determined by qRT-PCR.a, b and c represent independent biological replicates. Data represent means of technical replicates±s.e.m. ( n =6); *** P ≤0.001 and * P ≤0.05, significantly different from FN grown plants according to REST © 70 . ( b ) Primary root length of 7-day-old wild-type and ala10 seedlings grown on phosphate-depleted media. Data represented as box plot with marked median±s.d. ( n =115–165 from three biological replicates); *** P ≤0.001, significantly different with respect to wild type (WT) according to Mann–Whitney U -test. ( c ) Primary root length of 7- day-old wild-type and ala10 seedlings grown on phosphate-depleted media with the addition of liquid medium±lysoPC. Data represented as box plot with marked median±s.d. ( n =115–165 from three biological replicates); ** P ≤0.01, significantly different with respect to treatment without lysoPC according to Mann–Whitney U -test. Full size image ALA10 internalizes lysoPC and affects stomatal conductance Having established a function for ALA10 in the root, we investigated its role in guard cells. Strikingly, the stomatal conductance and transpiration rate in all three ala10 -knockout lines were remarkably lower than those of the wild type, both during day and night ( Fig. 7a ), whereas the net rate of photosynthesis was not affected ( Fig. 7a ). We next screened for cellular uptake of NBD-PC and -lysoPC in leaves following immersion of wild-type seedlings into liquid medium containing these compounds. Uptake of both compounds was readily observed in wild-type guard cells ( Fig. 7b , Supplementary Fig. 6a ). Not all wild-type guard cells took up the labelled phospholipids and in some cases the fluorescent signal was restricted to parts of the cell facing the stomatal pore ( Fig. 7b , Supplementary Fig. 6a , lower panels). NBD-lysoPC was also taken up into the guard cells of the ala10 mutants, but the amount of NBD-lysoPC uptake was significantly decreased in the ala10 mutants compared with the wild type ( Fig. 7c ), whereas a similar decrease in the uptake of NBD-PC was not observed in the mutant lines ( Supplementary Fig. 6b ). Also, the number of NBD-stained guard cells was significantly lower in the leaves of the mutant lines than in those of the wild type, but varied between the lines ( Fig. 7d , Supplementary Fig. 6c ). Although we were not able to carry out GUS reporter gene staining in the same cells as those used for the NBD-phospholipid uptake experiments, the fraction of guard cells in wild-type leaves that contributed to the uptake of labelled NBD-PC and -lysoPC (less than 50%) corresponds roughly to the fraction of cells that express GUS ( Fig. 7e ). 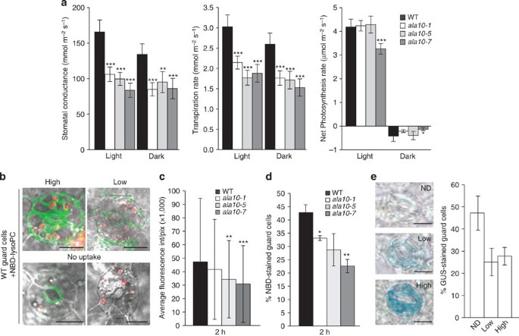Figure 7: ALA10 regulates stomatal conductance and internalizes lysoPC in guard cells. Physiological parameters were measured during the day and night for 7-week-old wild-type (WT) andala10-knockout plants. (a) Stomatal conductance, transpiration rate and net photosynthesis rate. Data represent means±s.d. (n=5–12); ***P≤0.001, **P≤0.01 and *P≤0.05, significantly different with respect to the WT according to Student’st-test. Three independent experiments were carried out with identical results. (b) Five-day-old wild-type orala10-knockout seedlings were incubated for 2 h in the presence of NBD-lysoPC and analysed by confocal microscopy. Representative overlays of fluorescence (NBD in green; chlorophyll in red) and bright field images of stained WT guard cells. Scale bar, 10 μm. High, example of guard cells characterized as high uptake capacity; low, example of guard cells characterized as low uptake capacity; no uptake, examples of guard cells classified as incapable of uptake (no staining or staining only in stomatal pore). (c) Quantification of NBD-lysoPC uptake by guard cells. Data represent means±s.d. (n=84–162 from three biological replicates), ***P≤0.001 and **P≤0.01, significantly different with respect to WT according to Student’st-test. (d) Number of NBD-lysoPC-stained guard cells. Data represent means±s.d. (n=682–781 from three biological replicates), **P≤0.01 and *P≤0.05 significantly different with respect to the WT according to Student’st-test. (e) Stained guard cells of 5-day-old plants expressing thepALA10-GUSconstruct. Data represent means±s.d. (n=6 leaves from a total of three plants). ND, not detectable. Scale bar, 10 μm. Figure 7: ALA10 regulates stomatal conductance and internalizes lysoPC in guard cells. Physiological parameters were measured during the day and night for 7-week-old wild-type (WT) and ala10 -knockout plants. ( a ) Stomatal conductance, transpiration rate and net photosynthesis rate. Data represent means±s.d. ( n =5–12); *** P ≤0.001, ** P ≤0.01 and * P ≤0.05, significantly different with respect to the WT according to Student’s t -test. Three independent experiments were carried out with identical results. ( b ) Five-day-old wild-type or ala10 -knockout seedlings were incubated for 2 h in the presence of NBD-lysoPC and analysed by confocal microscopy. Representative overlays of fluorescence (NBD in green; chlorophyll in red) and bright field images of stained WT guard cells. Scale bar, 10 μm. High, example of guard cells characterized as high uptake capacity; low, example of guard cells characterized as low uptake capacity; no uptake, examples of guard cells classified as incapable of uptake (no staining or staining only in stomatal pore). ( c ) Quantification of NBD-lysoPC uptake by guard cells. Data represent means±s.d. ( n =84–162 from three biological replicates), *** P ≤0.001 and ** P ≤0.01, significantly different with respect to WT according to Student’s t -test. ( d ) Number of NBD-lysoPC-stained guard cells. Data represent means±s.d. ( n =682–781 from three biological replicates), ** P ≤0.01 and * P ≤0.05 significantly different with respect to the WT according to Student’s t -test. ( e ) Stained guard cells of 5-day-old plants expressing the pALA10-GUS construct. Data represent means±s.d. ( n =6 leaves from a total of three plants). ND, not detectable. Scale bar, 10 μm. Full size image Identifying an active transport system for phospholipid uptake in plants is a rather unexpected finding and it is intriguing to ponder the physiological function of this system. In animal cells, plasma membrane P4-ATPases clear the outer leaflet of PS, which is an apoptotic signal [27] , [28] . A similar function is unlikely for ALA10, as plants do not have a surface-based mechanism for the recognition and removal of dying cells. Furthermore, ALA10 transports a variety of glycerophospholipids in addition to PS, including lysoPC ( Fig. 4d ). In the yeast S. cerevisiae , the two plasma membrane-localized P4-ATPases, Dnf1p and Dnf2p, have been proposed to be involved in endocytosis [29] . However, deletion of ALA10 did not cause any change in the rate of endocytosis as judged from internalization of an endocytotic marker ( Fig. 5d ). In the root tip, we may consider at least three possible functions for ALA10. First, the uptake of phospholipids from decaying humus could provide the roots with an alternative source of energy [30] . A lipid uptake system in roots would allow for the utilization of an energy supply other than the sun. While this is a controversial idea, the root is de facto a heterotrophic organ with the growing tip being the most metabolically active part. The fact that phospholipids internalized by ALA10 are rapidly metabolized by the plant cell ( Fig. 5b ), rather than ending up as passive membrane constituents, is in congruence with this possibility. Second, the desired portion of phospholipids may not be the energy-rich acyl chain but rather the phosphate group. Phosphate is a major growth-limiting factor for plants and internalization of phospholipids could contribute to phosphate uptake [31] . In this context, ALA10 could also function as a sensor of phospholipids in the soil environment that initiates signalling events leading to secretion of phosphatases. Like transceptors [32] , [33] , ALA10 is subject to phosphorylation in planta at serine and threonine residues [20] , [21] , which suggests that it is subject to tight regulation. One of the first signs of phosphate starvation in A. thaliana is that the root enters a determinate developmental programme in which primary root growth is arrested and cell differentiation is promoted, thereby stimulating lateral root growth and increasing the root surface area [34] . Notably, in response to phosphate starvation, the roots of the ala10 mutant were longer than those of the wild type ( Fig. 6b,c ). This finding suggests that ALA10 is part of the developmental programme that senses and responds to phosphate starvation, and its absence causes primary root growth to continue in the mutant plants even under phosphate-depleted conditions. Third, it is noteworthy that extracellular lysoPC is the product of PC degradation by secreted phospholipase A 2 (refs 35 , 36 , 37 ) and has recently been described as a signalling molecule in both symbiotic and pathogenic interactions between plants and microorganisms [36] , [38] , [39] . In the animal body, lysoPA produced extracellularly in response to various signals is internalized by an unknown mechanism before binding to intracellular targets [40] , [41] . In plants, lysoPC may also act intracellularly, as it has been shown to affect the cytoplasmically located autoinhibitory domain of the plasma membrane H + -ATPase [42] , [43] . Thus, ALA10 could be a lysoPC scavenger that internalizes this compound before it induces cellular responses. Whereas all three possibilities above may be considered, it is difficult to envision a role for ALA10 in acyl chain and phosphate uptake in stomatal guard cells, as these are rich in chloroplasts and are not growing parts of the plants. This argues against a specific need for energy and phosphate in these cells. However, several lines of evidence suggest that lysoPC has a signalling role in guard cells. LysoPC is involved in the light-induced signalling cascade, which leads to opening of the stomatal pore [44] . Although the underlying molecular mechanism is unknown, lysoPC is a specific activator of the plasma membrane H + -ATPase [42] , [45] , a proton pump that energizes the transport processes that lead to swelling of guard cells, which is a prerequisite for stomatal pore opening [46] . A role for lysoPC in cellular communication in the leaf has not been proposed before, but our results open up the possibility that lysoPC is involved in cell-to-cell signalling in a process mediated by ALA10. The stomatal pore is an entry point into the plant for pathogenic microorganisms [47] , [48] that secrete phospholipases that generate lysoPC and by doing so may trigger the opening of stomata [49] before invasion. Finally, it is also a possibility that in guard cells ALA10 might play a role in establishing and maintaining lipid asymmetry, as suggested for P4-ATPases in other organisms [1] . It was previously reported that S. cerevisiae Dnf1p and Dnf2p flip lysoPC from the outer to the inner leaflet of the plasma membrane [50] . Likewise, in the protozoa Leishmania donovani , a plasma membrane P4-ATPase, LdMT, has been shown to internalize miltefosine, a structural lysoPC analogue [51] . However, the physiological functions of these activities remain unclear. Nevertheless, they demonstrate that P4-ATPase-catalysed uptake of lysophospholipids is a general feature of eukaryotic cells even in free-living unicellular organisms. Among the seven classes of plant, fungal and animal P4-ATPases discussed in this work, it is striking that members of at least four are localized to the plasma membrane (Classes 3, 5, 6 and 7) and at least two (Classes 3 and 7) are additionally implicated in lysophospholipid internalization. Their sequences and physiological properties not only suggests that these four classes have a common evolutionary origin and might be considered as a single supercluster, but also opens up the possibility that P4-ATPases, which so far have mainly been implicated in the secretory pathway, have major unknown functions at the cell surface. Phylogenetic analyses of P4-ATPases Sequences with significant homology (Expect value<e −30 ) to the well-characterized S. cerevisiae P4-ATPase Drs2p were first identified by searching for sequences in completed genomes in the NCBI protein database ( http://blast.ncbi.nlm.nih.gov/ ) that represented different stages in the evolution of plants, fungi and animals. P4-ATPases in this data set were identified by the presence of signature motifs characteristic for P4-ATPases using the online P-type ATPase Classifier ( http://octo3.bioxray.au.dk/pump-classifier ) [4] and by constructing phylogenetic trees for sequences in each genome together with the S. cerevisiae P-type ATPases using Phylogeny.fr ( http://phylogeny.lirmm.fr/phylo_cgi/simple_phylogeny.cgi ) [52] , which also allowed for identification and removal of duplicates. Most genomes are still draft versions in the databases, so often the predicted P4-type ATPases do not represent complete proteins. Partial sequences were removed following alignment using Muscle [53] . The resulting data set comprised 162 sequences from 27 genomes (including rabbit SERCA2b Ca 2+ -ATPase as an outlier). The evolutionary history was inferred using the maximum likelihood method based on the JTT matrix-based model [54] . Initial tree(s) for the heuristic search were obtained automatically by applying the Neighbor-Join and BioNJ algorithms to a matrix of pairwise distances estimated using the JTT model, and then selecting the topology with the superior log likelihood value. All positions containing gaps and missing data were eliminated. There were a total of 563 positions in the final data set. To obtain statistical support for the placement of nodes, bootstrap values were inferred from 500 replicates [55] . Evolutionary analyses were conducted in MEGA6 (ref. 56 ). Accession numbers are listed in Supplementary Table 1 . DNA cloning All PCRs carried out in this study were performed using Phusion High-Fidelity DNA Polymerase (ThermoFisher Scientifics Inc., Waltham, MA, USA) under standard conditions recommended by the manufacturer. For genomic DNA amplification, a 2% final concentration of dimethyl sulfoxide (DMSO) was added to the reaction mixture. In some cases, an overlapping PCR strategy was used. In these cases, the first round of PCR amplifications was carried out to obtain the desired overlapping fragments. In a second round, 1–2 μl of each of these PCR reactions was mixed and used as template with primers that amplify the full-length product. Primers used and plasmids generated in this work can be found in Supplementary Table 2 . Full-length ALA10 (At3g25610) was amplified by overlapping PCR using purified root complementary DNA (cDNA) from A. thaliana Col-0 as template and oli_1938, oli_1939, oli_2042 and oli_2043. The PCR product was cloned into the pJET1.2/blunt vector using the CloneJET PCR Cloning Kit (Life Technologies, Carlsbad, CA, USA) and into pENTR/D-TOPO using the pENTR/D-TOPO Cloning Kit (Invitrogen, Life Technologies), generating plasmids pMP3171 and pMP3228, respectively. To express ALA10 in yeast for functional complementation, two modified versions of the yeast expression vector pRS423-GAL [57] were created, pMP3156 and pMP3157. The new plasmids allow for the generation of untagged or N-terminally MARGSH 10 -tagged constructs, respectively. To construct these plasmids, the unique Dra III site of pRS423-GAL was eliminated by enzymatic digestion followed by treatment with T4-DNA polymerase and religation, generating pMP3198. The GAL1-10 promoter fusion contained in this vector was amplified using primer oli_2777 together with oli_2821 (pMP3156) or oli_2755 (pMP3157). ALA10 was subcloned into these plasmids after PCR amplification using oli_2838 and oli_2945 or oli_2946, respectively. A mutated version of ALA10 , ala10D430N , was generated by overlapping PCR using the primer pairs oli_2946 and oli_3643 and oli_3642 and oli_2838 and cloned into pCR4 Blunt-TOPO (Invitrogen, Life Technologies), generating pMP3910. ala10D430N was further subcloned by Sph I/ Sal I digestion and ligation into pMP3157, producing the pMP3912 plasmid. All clones were fully sequenced. Full-length ALA2 was PCR-amplified from an ALA2 -containing pENTR/D-TOPO vector [16] using oli_1968 and oli_2942 and cloned directly using Sph I/blunt restriction into pMP3157 to obtain pMP3395. To generate a MARGSH 10 -tagged version of ALA3, the gene was PCR-amplified from pMP2033 (ref. 15 ) using primers oli_1995 and oli_2783 and cloned into pCR4 Blunt-TOPO to generate plasmid pMP4669. A Eco RI/ Apa I fragment containing full length ALA3 was excised from this plasmid and cloned into pMP4062 (ref. 17 ) to render pMP4670. For expression of ALA10 in planta , a genomic DNA fragment corresponding to the full open reading frame (ORF), was amplified by PCR and cloned into plasmid pENTR/D-TOPO as described above. After full sequencing, the DNA insert was transferred to the binary plasmid pMDC45 (ref. 58 ) using Gateway technology (Invitrogen, Life Technologies), rendering plasmid pMP3955. For expression of GFP-ALA10 in yeast, a fragment corresponding to the GFP ORF fused to the first nine amino-acid residues of ALA10 was amplified from pMP3955 using oli_5100 and oli_5110. This fragment, which also contains a sequence that overlaps with the GAL1-10 promoter, was transformed into yeast together with linearized pMP3390 digested with Sph I. After homologous recombination, plasmids were isolated from yeast, amplified in Escherichia coli and sent for sequencing. The promoter of ALA10 was cloned as a short (2,389 bp upstream of the ATG start codon) and long (3,013 bp upstream of ATG) version. The promoter fragments were PCR amplified using oli_3741 in combination with oli_3799 and oli_3740, respectively. Both fragments were cloned into pENTR/D-TOPO as described above and fully sequenced, giving rise to pMP4177 and pMP4176, respectively. For fusion to the reporter gene GUS , the promoter fragments were subcloned into pMDC162 (ref. 58 ) using Gateway technology to generate pMP4181 and pMP4179, respectively. Yeast strains and growth conditions Functional complementation and lipid translocation assays were carried out using S. cerevisiae mutant strain ZHY709 ( MATα his3 leu2 ura3 met15 dnf1Δ dnf2Δ drs2::LEU2 (ref. 9 )) and strain BY4741 ( MATα his3 leu2 ura3 met15 ; EUROSCARF) was used as wild type. Yeast cells were transformed by the lithium acetate method [59] . Cells were grown overnight on YPD plates (1% yeast extract, 2% peptone, 2% glucose, 2% agar) at 30 °C and 4–5 μl cells were washed in 1 ml water, before resuspension in 1 ml 100 mM lithium acetate and 15-min incubation at 30 °C. After short centrifugation, the supernatant was removed and 360 μl of transformation mix (33% polyethylenglycol M w 3,350, 100 mM lithium acetate, 300 μg ml –1 salmon sperm DNA) and 200–300 ng plasmid were added. Cells were resuspended by 1 min vortexing and incubated at 42 °C for 30 min. Cells were spun down, resuspended in 100 μl water and plated on synthetic SD [60] plates (0.7% yeast nitrogen base, 2% glucose, 1 × synthetic drop out media lacking histidine and uracil (Sigma-Aldrich, St. Louis, MO, USA), 2% agar). For complementation assays, transformants were incubated in liquid SG medium (same as SD but with galactose instead of glucose) for 4 h and then diluted with water to 0.3 OD 600 ml –1 . Drops (5 μl) were spotted on SD (control) or SG (Induced) plates and incubated at 30 °C for 2–3 days or at 20 °C for 7 days. When indicated, 0.05 μg ml –1 papuamide B (Flintbox, Lynsey Huxham; www.flintbox.com ), 1.6 μM duramycin (Sigma-Aldrich, St. Louis, MO, USA) and 2.5 μg ml –1 miltefosine (hexadecylphosphocholine; Calbiochem, La Jolla, CA, USA) were added to the synthetic SG media. All experiments were repeated independently at least three times. The S. cerevisiae mutant strain ZHY709 was used for GFP-ALA10 cloning by homologous recombination (see above). For visualization, individual freshly transformed yeast colonies were inoculated on 1 ml liquid SG medium and grown for 16 h at 28 °C with 120 r.p.m. shaking. Yeast microsomal membrane preparation and immunodetection Fresh yeast transformants were inoculated in selective SD medium and grown for 24 h at 28 °C with 100 r.p.m. shaking, before inoculation into SG media at a 1/100 dilution. After another 24-h incubation period under the same conditions, cells were harvested by centrifugation at 3,000 g at 4 °C for 5 min, washed twice in ice-cold water and resuspended 1/1 (w/v) in homogenization buffer (45% glycerol, 200 mM Tris-HCl pH 7.5, 40 mM EDTA pH 8, 0.5 mM DTT, 0.5 μg ml –1 pepstatin A, 50 μM PMSF). Cells were lysed by addition of one volume ice-cold acid-washed glass beads (0.5 mm), followed by four cycles of 1 min vortex and 1 min rest on ice. Samples were diluted to a half with GTED20 (20% glycerol, 100 mM Tris-HCl pH 7.5, 1 mM EDTA pH 8, 1 mM DTT, 1 μg ml –1 pepstatin A, 100 μM PMSF) and centrifuged at 3,000 g at 4 °C for 10 min to eliminate glass beads and cell debris. Total microsomal membrane fractions were collected by centrifugation at 100,000 g at 4 °C for 1 h and homogenized in GTED20. For Western Blot, total proteins were precipitated in 10% tricholoroacetic acid, run on 10% denaturing polyacrylamide gels and transferred to nitrocellulose membranes. A mouse monoclonal anti-RGSH antibody (QIAGEN Nordic, Copenhagen, Denmark; catalogue number 34650) was used for detection at a 1:5,000 dilution. Bands were visualized with the 5-bromo-4-chloro-3-indolyl phosphate/nitroblue tetrazolium (BCIP/NBT) colour development substrate (Promega, Madison, WI, USA). Original blot scans can be found in Supplementary Fig. 7 . NBD-lipid uptake in yeast Palmitoyl-(NBD-hexanoyl)-PS (NBD-PS), palmitoyl-(NBD-hexanoyl)-PE (NBD-PE), palmitoyl-(NBD-hexanoyl)-phosphocholine (NBD-PC), palmitoyl-(NBD-hexanoyl)-phosphatidylglycerol (NBD-PG), palmitoyl-(NBD-hexanoyl)-phosphatidic acid (NBD-PA) and 1-NBD-dodecanoyl-2-hydroxy- sn -glycero-3-phosphocholine (NBD-lyso-PC) were from Avanti Polar Lipids (Birmingham, AL, USA). Palmitoyl-(NBD-hexanoyl)-diacylglycerol (NBD-DAG) was purified on thin layer chromatography plates (see below) after enzymatic conversion of NBD-PS using an A. thaliana root extract and quantitated spectrophotometrically by comparison with known amounts of NBD-PC using a Fluoromax-4 fluorimeter (excitation 470 nm, emission 535 nm; Horiba, Edison, NJ, USA). NBD-lipid stocks (10 mM for PS, PE and PC; for all others 4 mM) were prepared in DMSO. For NBD-lipid uptake experiments [16] , cells were grown overnight at 28 °C (100 r.p.m.) in selective SG medium to 0.2–0.5 OD 600 ml –1 . Cells (10 OD 600 ml –1 ) were incubated in the same medium with 24–60 μM NBD-lipids for 30 min at 30 °C with periodic mixing. Before analysis by flow cytometry or confocal microscopy, cells were washed three times in ice-cold selection media without galactose, but containing 2% sorbitol, 3% (w/v) bovine serum albumin, and 20 mM NaN 3 . Flow cytometry of NBD-labelled cells was performed on a Becton Dickinson FACSCalibur (San Jose, CA) equipped with an argon laser using Cell Quest software. One microliter of 1 mg ml –1 propidium iodide in water was added to 1 × 10 7 cells in 1 ml sterile-filtered water just before analysis. Thirty thousand cells were analysed without gating during the acquisition. Live cells were selected based on forward/side-scatter gating and propidium iodide exclusion. A histogram of the green fluorescence (NBD) of living cells was used to calculate the mean fluorescence intensity of total cells. Accumulation of NBD-lipids is given as the percentage fluorescence intensity relative to ZHY709 transformed with empty vectors. One hundred per cent corresponds to 43±29 arbitrary units (NBD-PC), 73±20 arbitrary units (NBD-PS), 27±6 arbitrary units (NBD-PE), 60±1 arbitrary units (NBD-PG), 48±5 arbitrary units (NBD-PA), 8±3 arbitrary units (NBD-DAG), and 71±45 arbitrary units (NBD-lysoPC) and values are given as means±s.d. of at least three independent experiments. Transient expression in tobacco epidermal leaf cells Subcellular localization experiments were carried out by transient expression in tobacco epidermal cells [16] . Agrobacterium tumefaciens strain C58C1 (ref. 61 ) was transformed by electroporation, and transformants were selected on YEP plates (1% yeast extract, 2% peptone, 1.5% agar) containing 25 μg ml –1 gentamicin and 50 μg ml –1 kanamycin. Transformants were grown overnight in 2 ml liquid YEP media, washed in infiltration solution (10 mM MgCl 2 , 100 μM 4′-Hydroxy-3’,5’-dimethoxyacetophenone) and used for infiltration using 3-week-old Nicotiana benthamiana plants. To facilitate high expression of recombinant proteins A. tumefaciens strains carrying the different constructs were co-infiltrated with a strain carrying the p19 gene encoding the viral p19 protein that specifically inhibits plant posttranscriptional gene silencing. When several constructs were co-infiltrated, all A. tumefaciens strains mixed were used to the same final concentration (0.03 OD 600 ml –1 ). Expression was visualized 4–5 days after infiltration. Plasmolysis of epidermal tobacco cells was achieved by infiltrating the leaves with a 1 M mannitol solution 1–2 min before sample preparation for confocal microscopy visualization. Plant transformation pALA10 - GUS constructs were introduced into wild-type A. thaliana by floral dipping [62] , using A. tumefaciens strain C58C1 (ref. 61 ), transformed as above. A 400-ml overnight A. tumefaciens culture in YEP medium was centrifuged at 6,000 g for 10 min at room temperature and resuspended in 200 ml sucrose solution (5% sucrose, 0.005% Silwet L-77). Flowers from 5–7-week-old plants soil-grown under long day conditions (16 h light, 8 h darkness) were dipped in the A. tumefaciens solution for 30 s and let to dry. The procedure was repeated three consecutive times with a week in between. Growth of A. thaliana For selection of transformed A. thaliana plants, seeds were selected on plates containing ½ Murashige and Skoog [63] (½MS) media including vitamins (Duchefa Biochemie; Amsterdam, The Netherlands), 0.5 g l −1 2-( N -morpholino)ethanesulfonic acid (MES) and 1% agar (A1296; Sigma Aldrich, St. Louis, MO, USA), buffered to pH 5.7 by the addition of KOH and supplemented with 25 μg ml –1 hygromycin solution. Seeds of A. thaliana corresponding to wild-type Col-0, transgenic promoter:GUS plants and mutant lines lacking ALA10 ( ala10-1 (SALK_024877) , ala10-5 (WiscDsLox_499E11) or ala10-7 (GABI_78G10)) were surface-sterilized and transferred to ½MS media. After a 3-day vernalization, plates were transferred to a growth chamber and incubated under a 12-h light regime with the following scheme: t =0 h, 20 °C, ≈40 μmol photons m –2 s –1 light intensity; t =3 h, 20 °C, ≈160 μmol photons m –2 s –1 light intensity; t =7 h, 22 °C, ≈85 μmol photons m –2 s –1 light intensity; t =10 h, 20 °C, ≈40 μmol photons m –2 s –1 light intensity; t =12 h, 20 °C, darkness; t =16 h, 17 °C, darkness; t =20 h, 15 °C, darkness; and t =22 h, 17 °C, darkness. Five-day-old seedlings were used in all experiments, unless otherwise stated. For the phenotypic screen and expression analysis of ALA10 under phosphate starvation, full nutrition (FN) medium [64] (2 mM KNO 3 , 1 mM NH 4 NO 3 , 1 mM glutamine, 3 mM KH 2 PO 4 /K 2 HPO 4 pH 5.8, 4 mM CaCl 2 , 1 mM MgSO 4 , 2 mM K 2 SO 4 , 3 mM MES pH 5.7, 0.5% (w/v) sucrose, 40 μM Na 2 FeEDTA, 60 μM H 3 BO 3 , 14 μM MnSO 4 , 1 μM ZnSO 4 , 0.6 μM CuSO 4 , 0.4 μM NiCl 2 , 0.3 μM HMoO 4 , 20 nM CoCl 2 ) was prepared with the addition of 1% agar. Medium without phosphate (NoP) contained all components as in FN except that KH 2 PO 4 /K 2 HPO 4 was replaced with 2.5 mM KCl. For lysoPC testing, 10 μl NoP medium supplemented with 200 μM lysoPC (1 mg lysoPC dissolved in 20 μl 70% ethanol) was spotted directly onto the root tip in three 24-h repeats, starting at day 4 after transfer to light. For control plants, the same amount of NoP medium supplemented with ethanol was used. Plants were photographed and root length measured at day seven after transfer to light. Expression analysis Plant material from 7-day-old wild-type seedlings grown under phosphate starvation (NoP) and under normal phosphate conditions (FN) was harvested and immediately frozen in liquid N 2 . RNA was purified from the root fraction using an E.Z.N.A Plant RNA Kit (Omega Bio-Tek, Norcross, GA, USA) following the manufacturer’s instructions. gDNA removal was carried out using DNA-free DNase Treatment & Removal reagents (Life Technologies). cDNA was generated using an iScript cDNA Synthesis Kit (BioRad, Copenhagen, Denmark). To monitor the expression level of ALA10 under phosphate starvation, real time-PCR using Brilliant II SYBR Green qPCR Master Mix (Agilent Technologies, Glostrup, Denmark) was performed [65] according to the maufacturer’s instructions. PCR was carried out using a Mx3000P (Stratagene, La Jolla, CA) real-time PCR system in 25-μl reactions containing 40 ng of cDNA, 10 pmol of each primer and a 1:1,000 diluted reference dye. A standard series made with serial diluted cDNA of known concentration was used to determine primer specificity and efficiency. PCR reactions were initiated with a 15-min denaturation step at 95 °C, followed by 40 cycles of 10 s at 95 °C, 30 s at 60 °C and 30 s at 72 °C and one final cycle of 1 min 95 °C, 1 min at 60 °C and 10 min at 95 °C, creating the dissociation curve. Fluorescence was detected after each cycle. Three independent biological replicates were analysed in triplicates with two technical replicates. ACTIN2 and UBC21 were used as reference genes. Gene-specific primers for reference genes and ALA10 are presented in Supplementary Table 2 . Leaf gas exchange measurements Wild-type Col-0 and ala10 -knockout seeds were vernalized for 3 days and grown in standard soil under an 8-h light regime (22 °C, 54% humidity, 8 h light/16 h darkness, photosynthetic photon flux density of ∼ 150 μmol photons m –2 s –1 ) for 7 weeks. Leaf gas exchange measurements were conducted [66] . A fully expanded leaf was placed in the cuvette of a CIRAS-2 portable photosynthesis and transpiration monitor (CIRAS-2 Potable Photosynthesis System; PP Systems, Amesbury, MS, USA). The concentration of CO 2 in the cuvette was maintained at 400 p.p.m., the humidity at 80% and the light intensity at 125 μmol photons m –2 s –1 . Fluorescent assays and GUS staining in planta To visualize lipid uptake in plants, 5-day-old seedlings were transferred to liquid ½MS medium (pH 5.7) exactly 2 h after the start of the light period. Following a preincubation at 25 °C for 5 min, NBD-lipid was added from a 10-mM stock in DMSO to a final concentration of 60 μM and the incubation was continued for the indicated periods. For experiments in roots, uptake was stopped by exchanging the lipid-containing medium with fresh ½MS containing 1% tergitol (NP-40, Sigma). Samples were washed twice for 5 min with ½MS liquid medium with detergent and once with medium lacking detergent, and kept in the dark in fresh ½MS medium at room temperature until confocal microscopy visualization. The same procedure was used for lipid uptake assays in guard cells, with the exception that seedlings were washed only once with ½MS medium without detergent. To monitor endocytosis, seedlings were harvested and incubated in ½MS medium as above but with the addition of FM4-64 (from a 32 mM DMSO stock) to a final concentration of 2 μM. After the indicated periods, plants were rinsed in water, mounted on microscope slides, and visualized by confocal microscopy. To determine the tissue-specific expression of ALA10 , independent plants for each GUS-expressing line were selected and intact seedlings were stained for GUS activity [67] . Samples were incubated in a 5-bromo-4-chloro-3-indolyl β-D-glucuronide (X-gluc) solution (3 mM K 3 (Fe(CN) 6 ), 3 M K 4 (Fe(CN) 6 ), 0.2% Triton-X-100, 50 mM KH 2 PO 4 /K 2 HPO 4 pH 7.2, 2 mM X-gluc) at 37 °C in the dark for the times specified. After incubation, samples were cleared in 96% ethanol. Microscopy visualization and quantification of fluorescence For analysis of GUS-expressing plants, a Nikon Eclipse 80i light microscope equipped with a Nikon Digital Sight DS L1 image-capture system was used. Depending on the size of the visualized area, a 4 × /0.10 numerical aperture (N.A. ), 10 × /0.30 N.A., 20 × /0.50 N.A. or 40 × /0.75 N.A. objective was used. A Leica SP2 UV MP or SP5 II spectral confocal laser scanning microscope (Leica Microsystems, Heidelberg, Germany) was used for fluorescence microscopy. For visualization of plant tissues, a 63 × /1.2 N.A. water immersion objective was used and all yeast imaging was done using a 100 × /1.40 N.A. oil immersion objective. In plants, both GFP and YFP were excited at 488 nm, and emission spectra were recorded between 490 and 508 nm for GFP (green channel) and 545 and 560 nm for YFP (magenta channel). Sequential scanning between lines was used to follow both fluorescent proteins at once. No fluorescence bleed-through of YFP or GFP signals was detected under our experimental conditions. For GFP-ALA10 visualization in yeast cells, GFP was excited at 488 nm and emission was recorded between 496 and 565 nm. To visualize internalized NBD-lipids in yeast cells and plant tissues, NBD was excited at 458 nm and emission signals were recorded between 495 and 550 nm for yeast and root tips and between 480 and 565 nm for guard cells. Autofluorescence of chloroplasts in guard cells was recorded between 647 and 695 nm. FM4-64 was excited at 514 nm and emission recorded between 700 and 760 nm. All fluorescent signals were quantified using ImageJ ( http://imagej.nih.gov/ij/ ). For quantification of NBD or FM4-64 signals, regions of interest (ROI) were defined for each image and average pixel intensity was measured in each region. For plant roots, the ROI enclosed the root tip right under the elongation zone. For guard cells, the ROI comprised both guard cells of each stomata. Only those stomata in which at least one guard cell showed clear fluorescence at internal membranes were considered as competent for uptake. Analysis of NBD-lipid metabolism in yeast and plants Following NBD-lipid uptake assays in yeast, total cellular lipids were extracted twice from 100 μl of cell suspension in two volumes of chloroform/methanol 1/1 (v/v) [68] . For plants, 10-15 NBD-lipid-labelled seedlings were ground, resuspended in 100 μl ½MS media and extracted twice as above. The lipid containing chloroform/methanol phase was collected, dried and resuspended in a small volume of chloroform before separation by thin-layer chromatography using chloroform/ethanol/water/triethylamine (30/35/7/35, v/v/v/v; ref. 69 ). NBD-lipid standards were chromatographed on the same plate. Fluorescent lipid spots were visualized with a Typhoon Trio Variable Mode Imager (GE Healthcare, Brøndby, Denmark). For preparation of root extracts, the roots from 10–15 5-day-old seedlings were cut and ground in the presence of ½MS medium (pH 5.7), before addition of NBD-lipids and incubation as indicated for whole seedlings above. After incubation, samples were centrifuged shortly to remove debris and the supernatant was collected for total lipid extraction. Original thin-layer chromatography scans can be found in Supplementary Figs 8 and 9 . Statistical analyses For statistical analysis of real time-PCR data, the programme REST-384 was used ( http://www.gene-quantification.de/download.html#rest-384 ; ref. 70 ). The primary root length data were analysed using the Mann–Whitney U -test ( http://elegans.som.vcu.edu/~leon/stats/utest.html ), while statistical analyses for NBD-lipid uptake in yeast and plants and stomatal conductance were performed using a Student’s t -test, with a two-tailed distribution and two-sample unequal variance. How to cite this article: Poulsen, L. R. et al . A phospholipid uptake system in the model plant Arabidopsis thaliana . Nat. Commun. 6:7649 doi: 10.1038/ncomms8649 (2015).